The NCA sodium leak channel is required for persistent motor circuit activity that sustains locomotion Persistent neural activity, a sustained circuit output that outlasts the stimuli, underlies short-term or working memory, as well as various mental representations. Molecular mechanisms that underlie persistent activity are not well understood. Combining in situ whole-cell patch clamping and quantitative locomotion analyses, we show here that the Caenorhabditis elegans neuromuscular system exhibits persistent rhythmic activity, and such an activity contributes to the sustainability of basal locomotion, and the maintenance of acceleration after stimulation. The NALCN family sodium leak channel regulates the resting membrane potential and excitability of invertebrate and vertebrate neurons. Our molecular genetics and electrophysiology analyses show that the C. elegans NALCN, NCA, activates a premotor interneuron network to potentiate persistent motor circuit activity and to sustain C. elegans locomotion. Collectively, these results reveal a mechanism for, and physiological function of, persistent neural activity using a simple animal model, providing potential mechanistic clues for working memory in other systems. Animals generate sustained responses to transient sensory stimuli [1] . The ability to sustain neural activity upon brief stimulation is crucial for animal survival, for example, by allowing them to both initiate and sustain the escape response after they are briefly surprised or threatened. Single unit recordings from the primate prefrontal cortex neurons detected sustained neuronal firing during the late phase of a delayed response task [2] , [3] . Since these initial findings, persistent neural activities that outlast the input stimuli have been found in multiple brain regions, and implicated in working memory and motor planning [4] , [5] , [6] , [7] . For example, in the hippocampus, persistent neural activity underlies the auditory working memory [8] , [9] . In the brainstem, it controls head and eye movements [10] . Deficits in persistent neural activity have been associated with schizophrenia, attention deficit hyperactivity disorder and stress [11] , [12] . Current studies suggest that persistent neural activity may result from either reverberant network activity, or, individual neurons sustained by their intrinsic biophysical properties. The excitatory alpha-amino-3-hydroxy-5methyl-4-isoxazole propionic acid [13] , [14] and N-methyl-D-aspartate (NMDA) receptors [15] , [16] , [17] , as well as the inhibitory gamma-aminobutyric acid (GABA) receptors [18] , [19] , contribute to the reverberant network-dependent persistent activity. Conductance wise, the L-type Ca 2+ channel (Cav1.3) and calcium-activated nonspecific cation channels (CANs) have been implicated in persistent activity sustained by the intrinsic property of individual neurons. The CAN currents that sustain neuronal activities share physiological properties of slow depolarization with slow or no inactivation [20] . Pharmacological activation of some metabotropic cholinergic receptors, which activates CAN currents, induces persistent neural activity in the prefrontal cortex [21] , the hippocampus [22] , the entorhinal cortex [23] and the lateral amygdala [24] . Canonical transient receptor potential channels (TRPCs) have been proposed to underlie some CAN currents [25] , [26] , [27] . The lamprey reticulospinal neurons sustain action potential firing after a brief tap on the snout, which induces an escape response; the sustained neural activity requires CAN currents activated by the NMDA receptors [15] , [28] . Moreover, serotonin- or voltage-activated persistent Na + currents have been implicated in regulating neuronal bi-stability that may associate with the persistent activity in motor neurons [29] , [30] . Despite the prevalence of persistent activity in a variety of brain areas and across species, as well as its physiological relevance to learning, memory and mental disorders [31] , molecular identities of most CAN channels that underlie such an activity remain unknown. Recently, we and others identified a conserved sodium (Na + ) leak channel, namely NALCN in vertebrates and NCA in invertebrates [32] , [33] , [34] , [35] , [36] , [37] . Mutations in human NALCN have been associated with a spectrum of physiological impairments, including severe hypotonia, speech impairment, growth failure and cognitive delay [38] , [39] . The NALCN/NCA channel is a voltage-independent, Tetrodotoxin (TTX)-insensitive and substance P-potentiated constitutive Na + -permeable channel [34] , [40] . Its absence leads to the hyperpolarization of mouse hippocampal and cortical neurons [34] , [40] , Caenorhabditis elegans premotor interneurons [37] and snail respiratory pacemaker neurons [36] , revealing its conserved role in establishing neuronal resting membrane potential. NALCN is ubiquitously expressed in the mouse nervous system. Nonconditional NALCN knockout mice exhibit severely disrupted respiratory rhythm and lethality within 24 h after birth [34] . The role of NALCN in the mature brain remains unknown. Interestingly, the neuromodulator substance P facilitates the occurrence of post-stimulus discharges, and potentiates TTX-independent plateau potential in the turtle spinal neurons [41] , suggesting that the NALCN channel may also regulate persistent neural activity. In C. elegans , the loss of NCA channel activity leads to abrupt and frequent stops in movements [35] . These results suggest that, in addition to contributing to the resting membrane potential, NCA may regulate motor circuit activity that sustains locomotion. In this study, we report the detection of persistent rhythmic motor circuit activity in the C. elegans neuromuscular preparation. In the absence of the NCA channel, the persistent motor circuit activity is abolished, coinciding with an unsustained locomotion under both spontaneous and evoked conditions. A specific restoration of the NCA channel in premotor interneurons is sufficient to restore the persistent motor circuit activity, as well as the motor deficit. These results suggest that the NCA Na + leak channel, mainly through premotor interneurons, is required for the persistent motor circuit activity that sustains locomotion. A C. elegans preparation exhibits persistent rhythmic activity A C. elegans electrophysiology preparation was developed [42] , modified and optimized in recent years, including the adaption of optogenetic stimulation of sensory, motor and premotor interneurons [43] , [44] , [45] , [46] , to allow for quantitative assessment of the physiological properties of the C. elegans motor system. Collectively, these studies determined that the C. elegans musculatures receive excitatory cholinergic inputs to activate calcium-driven action potential bursts in body wall muscles and sustained muscle contraction, whereas inhibitory GABAergic inputs lead to the hyperpolarization of the muscle membrane potential, inhibition of action potential firing and muscle relaxation. The physiological nature of pre- and post-synaptic communication remains unsettled; however, current studies pointed towards the presence of graded postsynaptic currents (PSCs) at the neuromuscular junctions [47] . PSC bursts, consisted of high-frequency miniature postsynaptic currents (mPSCs), were occasionally observed in nascent preparations when dissected animals were less fixed [46] . Bursts of PSCs with further increased mPSC frequencies were more readily observed upon the stimulation of cholinergic motor neurons and premotor interneurons [46] . To characterize the physiological properties of the C. elegans motor circuit, we performed prolonged recordings of the dissected young adult preparations, using conditions that we and others optimized for observing consistent action potential firing by body wall muscles [44] , [48] (Methods). In wild-type preparations, in the absence of any form of stimulations, we consistently observed, at low frequency (~10% of preparations), trains of spontaneous fast rhythmic PSC bursts. These events, which we termed rhythmic PSC bursts (rPSCs), were distinct from the reported high-frequency mPSC events ( Supplementary Fig. 1 ). Unlike the reported spontaneous and stimulated mPSC bursts [43] , [46] , spontaneous rPSCs consist of a train of rhythmic depolarization events of ~50–300 pA at 3–7 Hz, which often lasted ~3–10 s ( Supplementary Fig. 1 ). These patterned rhythmic depolarization events were robustly evoked (in ~90% preparations) when multiple premotor interneurons were stimulated by ChR2, whereas the activation of a single premotor interneuron pair AVA sufficiently, although less effectively (in ~70% preparations), evoked similar events ( Fig. 1 , Supplementary Fig. 2 ). Using current clamp at the same body wall muscles, we confirmed that these rPSCs were tightly associated with the burst firing of action potentials ( Fig. 1 , Supplementary Fig. 2 ). The rPSCs thus resemble patterned physiological neural network activity. 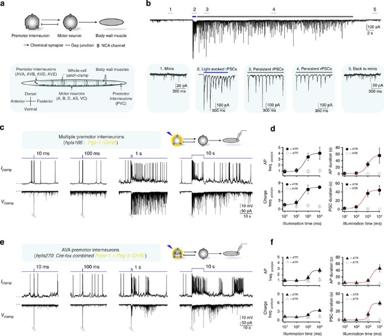Figure 1: The neuromuscular preparation exhibits persistent activity. (a; Upper panel) A simplified schematic of theC. elegansadult motor circuit components and connectivity58. The hexagon, circle and oval represent premotor interneurons, excitatory motor neurons and body wall muscles, respectively; the arrow and lines denote chemical synapses and gap junctions, respectively, with the arrowhead pointing towards the postsynaptic neurons. The NCA channel is expressed in premotor interneurons and excitatory motor neurons. (Lower panel) A diagram of the anatomic organization of theC. elegansneuromuscular system. Colour codes denote different neuronal groups (black: premotor interneurons and excitatory motor neurons that potentiate backward locomotion; dark grey: premotor interneurons and excitatory motor neurons that potentiate forward locomotion; light grey: inhibitory and other motor neurons; light blue: body wall muscles). Recordings were performed on the anterior ventral body wall muscles (muscle nos 9–14). (b) A sample trace of rPSCs and persistent rPSCs evoked by 1-s blue LED light stimulation of multiple neurons that include several premotor interneurons (hpIs166;Pglr-1::ChR2). Lower panels provide enlarged view of the indicated regions (dash lines 1–5). (c) Representative traces evoked by the blue LED light illumination with different durations inhpIs166animals, under current (Iclamp) and voltage clamp (Vclamp) configuration. Blue lines denote the stimulation protocol. The upper right panel illustrates the ChR2 loci in the motor circuit (yellow) and position of recording electrode. (d; Upper left panel) the ratio between the frequency of body wall muscle action potentials (APs) post- and pre-blue light illumination, with or without ATR; (upper right panel) the duration of the elevated APs firing post-stimulation; (lower left panel) the ratio between the rPSCs charge post- and pre-blue light illumination; (lower right panel) duration of increased rPSCs.Vclamp: 10 ms (n=10), 100 ms (n=7), 1 s (n=12), 10 s (n=10);Iclamp: 10 ms (n=14), 100 ms (n=9), 1 s (n=14), 10 s (n=7). (e) Sample traces evoked by the same illumination protocol inhpIs270(Cre-loxPnmr-1+rig-3::ChR2) animals, where AVA is specifically activated among premotor interneurons. (f) Quantifications fore. Muscles were held at 0 pA inIclampand at −60 mV inVclamp, respectively.Vclamp: 10 ms (n=7), 100 ms (n=6), 1 s (n=10), 10 s (n=14);Iclamp: 10 ms (n=11), 100 ms (n=7), 1 s (n=11), 10 s (n=9). Error bars, s.e.m. Data were collected from more than six biological and technical replicates (independent culture preparations). SeeSupplementary Figs 1–3. Figure 1: The neuromuscular preparation exhibits persistent activity. ( a ; Upper panel) A simplified schematic of the C. elegans adult motor circuit components and connectivity [58] . The hexagon, circle and oval represent premotor interneurons, excitatory motor neurons and body wall muscles, respectively; the arrow and lines denote chemical synapses and gap junctions, respectively, with the arrowhead pointing towards the postsynaptic neurons. The NCA channel is expressed in premotor interneurons and excitatory motor neurons. (Lower panel) A diagram of the anatomic organization of the C. elegans neuromuscular system. Colour codes denote different neuronal groups (black: premotor interneurons and excitatory motor neurons that potentiate backward locomotion; dark grey: premotor interneurons and excitatory motor neurons that potentiate forward locomotion; light grey: inhibitory and other motor neurons; light blue: body wall muscles). Recordings were performed on the anterior ventral body wall muscles (muscle nos 9–14). ( b ) A sample trace of rPSCs and persistent rPSCs evoked by 1-s blue LED light stimulation of multiple neurons that include several premotor interneurons ( hpIs166 ; Pglr-1 ::ChR2). Lower panels provide enlarged view of the indicated regions (dash lines 1–5). ( c ) Representative traces evoked by the blue LED light illumination with different durations in hpIs166 animals, under current ( I clamp ) and voltage clamp ( V clamp ) configuration. Blue lines denote the stimulation protocol. The upper right panel illustrates the ChR2 loci in the motor circuit (yellow) and position of recording electrode. ( d ; Upper left panel) the ratio between the frequency of body wall muscle action potentials (APs) post- and pre-blue light illumination, with or without ATR; (upper right panel) the duration of the elevated APs firing post-stimulation; (lower left panel) the ratio between the rPSCs charge post- and pre-blue light illumination; (lower right panel) duration of increased rPSCs. V clamp : 10 ms ( n =10), 100 ms ( n =7), 1 s ( n =12), 10 s ( n =10); I clamp : 10 ms ( n =14), 100 ms ( n =9), 1 s ( n =14), 10 s ( n =7). ( e ) Sample traces evoked by the same illumination protocol in hpIs270 (Cre-lox Pnmr-1 + rig-3 ::ChR2) animals, where AVA is specifically activated among premotor interneurons. ( f ) Quantifications for e . Muscles were held at 0 pA in I clamp and at −60 mV in V clamp , respectively. V clamp : 10 ms ( n =7), 100 ms ( n =6), 1 s ( n =10), 10 s ( n =14); I clamp : 10 ms ( n =11), 100 ms ( n =7), 1 s ( n =11), 10 s ( n =9). Error bars, s.e.m. Data were collected from more than six biological and technical replicates (independent culture preparations). See Supplementary Figs 1–3 . Full size image We consistently observed the reoccurrence of rPSCs after the termination of optogenetic stimulation of multiple premotor interneurons ( hpIs166 , Fig. 1a ). These events, which we termed persistent rPSCs, were typically observed within 30–40 s after the 1-s stimulation, before the preparation resumed to frequent mPSCs without an organized pattern ( Fig. 1b ). A longer (10 s) stimulation evoked longer duration of persistent rPSCs ( Fig. 1c,d ). Persistent rPSCs were also reliably observed after either 1- or 10-s stimulation of a single premotor interneuron pair AVA ( hpIs270 , Fig. 1e,f ). Neither evoked rPSCs nor persistent rPSCs were observed when animals cultured without all- trans retinal (ATR), a co-factor for ChR2 activation, were photostimulated by the same protocol ( Supplementary Fig. 3 ). Some preparations exhibited a delay in the onset of persistent rPSCs, which may result from either a requirement for synaptic vesicle replenishment or negative feedback after strong stimulation. The presence of persistent rPSCs suggests that the C. elegans motor circuit, similar to neural networks in other animals [31] , has the ability to generate persistent neural activity. nca(lf) sodium leak channel mutants cannot sustain locomotion If persistent rPSCs play a role in motor behaviours, mutations that affect the C. elegans’ motor pattern may provide clues to molecular mechanisms that regulate persistent rPSCs. We examined potential requirement of several cation channels that were implicated in C. elegans neuronal activity and motor behaviours; one such candidate is the Na + leak channel NCA. Previously, we and others have showed that NCA is required for proper motor patterns both on solid media and in liquid [32] , [33] , [35] , [37] , [49] . nca(lf) , the loss of function ( lf ) mutants for functionally redundant NCA channel subunits, NCA-1 and NCA-2, and nlf-1 , the lf mutants for an endoplasmic reticulum protein that specifically facilitates the membrane delivery of the NCA channel [37] , are fainters , named initially after their hypersensitivity to halothane [50] . Qualitatively, fainters stay more frequently in an idle mode than wild-type animals under standard culture conditions [37] ; they are however fully capable of active locomotion, briefly or in long period, upon brief or sustained sensory stimulation (for example, touch or starvation) [35] , [51] . To quantify the behavioural differences between wild-type and nca(lf) animals, we re-examined their motor behaviours using an automated tracking microscope at high temporal resolution. We first focused on the continuity of spontaneous basal movement for animals in explorative mode (Methods)—movements in the same directions ( Fig. 2a ), represented as the distribution of duration ( Fig. 2b ), the mean duration (Upper panel, Fig. 2c ) and frequency of transition between forward and backward movements (Lower panel, Fig. 2c ). Under the same condition (Methods), consistent with previous reports, nca(lf) mutants exhibited a specific loss of forward and backward movements of long duration when compared with wild-type animals ( Fig. 2b,c ). However, a previously unreported, more telling observation, was that these animals exhibited a drastic, approximately fivefold increase in short duration in both forward and backward movements ( Fig. 2b ) that coincided with a similar fold increase in re-initiation of movements (Lower panel, Fig. 2c ). These phenotypes suggest that fainters are capable of initiating locomotion, but fail to sustain it. Their ‘idleness’ ( Supplementary Fig. 4 ) thus consists of short movements accompanied by high-frequency pause and re-initiation of movements ( Fig. 2 ; Supplementary Movie 1 ). Similar behavioural deficiencies in motor patterns were observed for nlf-1 mutants ( Supplementary Figs 4 and 5 ). These results support a specific requirement of the NCA channel in sustaining locomotion. 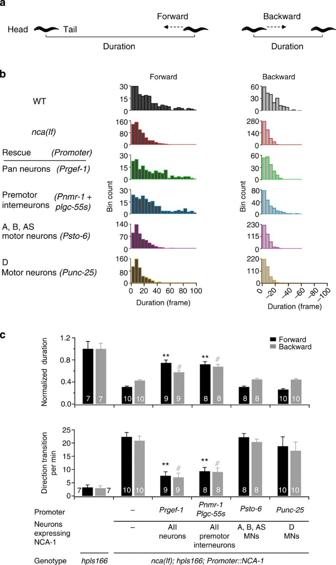Figure 2: CA sodium leak channel is required to sustain locomotion. (a) A schematic of the forward and backward movement inC. elegans. (b) Histograms of the duration of directional movement of animals on plates (see Methods). Left panels, forward locomotion; right panels, backward locomotion. The duration here was represented by the number of video frames (100 ms per frame) during each period of directional movements. The duration of both forward and backward movements was significantly reduced innca(lf)mutants; this defect was significantly rescued by restoring expression of NCA in all premotor interneurons (Pnmr-1+Plgc-55s), but not in excitatory (Psto-6) or inhibitory (Punc-25) motor neurons. Note that bin counts (yaxis) were substantially increased innca(lf)animals, and reduced when NCA-1 was restored in premotor interneurons. All animals hadhpIs166;hpIs166was treated as wild-type for this set of experiment. (c) Quantifications of the average duration (upper) and frequency of directional change (lower) of the same set of animals. **P<0.01, #P<0.05, againstnca(lf)mutants by the Mann–WhitneyU-test. Error bars, s.e.m. Data were collected from more than three biological and technical replicates (independent culture preparations). SeeSupplementary Figs 4 and 5,Supplementary Movie 1. Figure 2: CA sodium leak channel is required to sustain locomotion. ( a ) A schematic of the forward and backward movement in C. elegans . ( b ) Histograms of the duration of directional movement of animals on plates (see Methods). Left panels, forward locomotion; right panels, backward locomotion. The duration here was represented by the number of video frames (100 ms per frame) during each period of directional movements. The duration of both forward and backward movements was significantly reduced in nca(lf) mutants; this defect was significantly rescued by restoring expression of NCA in all premotor interneurons ( Pnmr-1 + Plgc-55s ), but not in excitatory ( Psto-6 ) or inhibitory ( Punc-25 ) motor neurons. Note that bin counts ( y axis) were substantially increased in nca(lf) animals, and reduced when NCA-1 was restored in premotor interneurons. All animals had hpIs166 ; hpIs166 was treated as wild-type for this set of experiment. ( c ) Quantifications of the average duration (upper) and frequency of directional change (lower) of the same set of animals. ** P <0.01, # P <0.05, against nca(lf) mutants by the Mann–Whitney U -test. Error bars, s.e.m. Data were collected from more than three biological and technical replicates (independent culture preparations). See Supplementary Figs 4 and 5 , Supplementary Movie 1 . Full size image The NCA channel activity is required for persistent rPSCs NCA’s specific role in sustaining locomotion implies potential requirement of the Na + leak channel in persistent rPSCs. Indeed, while an activation of premotor interneurons by ChR2 resulted in similar evoked rPSCs between wild-type animals and nca(lf) mutants during stimulation ( Supplementary Fig. 6 ), no persistent rPSCs were observed in nca(lf) mutants after stimulation ( Fig. 3a,c ; Supplementary Fig. 7a ). Consistently, no persistent action potential firings were observed in nca(lf) mutants ( Fig. 3b,d ; Supplementary Fig. 7b ). 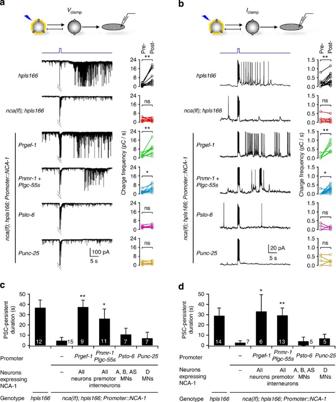Figure 3: Persistent motor circuit activity requires the NCA channel. (a) RepresentativeVclamptraces before, during and after 1s-blue light stimulation via thehpIs166transgene in various genetic backgrounds. Right panels, discharge frequency before and after the blue light stimulation. Connected lines denote recordings from the same preparation. (b) RepresentativeIclamptraces before, during and after 1s-blue light stimulation in various genetic backwards. (c) Quantification of the duration of persistent rPSCs post stimulation. (d) Quantification of the duration of persistent action potential firing post stimulation. Muscles were held at −60 mV inVclampand at 0 pA inIclamp, respectively. *P<0.05, **P<0.01, againstnca(lf)mutants by the Mann–WhitneyU-test. Error bars, s.e.m. Data were collected from more than five biological and technical replicates (independent culture preparations). SeeSupplementary Figs 6–8. Figure 3: Persistent motor circuit activity requires the NCA channel. ( a ) Representative V clamp traces before, during and after 1s-blue light stimulation via the hpIs166 transgene in various genetic backgrounds. Right panels, discharge frequency before and after the blue light stimulation. Connected lines denote recordings from the same preparation. ( b ) Representative I clamp traces before, during and after 1s-blue light stimulation in various genetic backwards. ( c ) Quantification of the duration of persistent rPSCs post stimulation. ( d ) Quantification of the duration of persistent action potential firing post stimulation. Muscles were held at −60 mV in V clamp and at 0 pA in I clamp , respectively. * P <0.05, ** P <0.01, against nca(lf) mutants by the Mann–Whitney U -test. Error bars, s.e.m. Data were collected from more than five biological and technical replicates (independent culture preparations). See Supplementary Figs 6–8 . Full size image nlf-1 mutants exhibited similar persistent rPSCs defects: they responded to premotor interneuron stimulation with similar depolarization patterns as wild-type animals ( Supplementary Fig. 6 ); there was however a specific loss of persistent rPSCs and action potential firings post stimulation ( Supplementary Fig. 8 ). A specific defect in persistent rPSCs, with normal evoked transient rPSCs, was unique for nca(lf) and nlf-1 mutants, and was not observed in other cation channel mutants such as VGCC/egl-19(lf) (data not shown). These results indicate that the Na + leak channel NCA may be specifically required for persistent rPSCs. Premotor interneurons are required for persistent rPSCs The high frequency of brief movements exhibited by both nca(lf) and nlf-1 mutants corresponds with a previously unexplained calcium imaging phenotype of the C. elegans premotor interneurons AVA and AVE. These interneuron pairs, which provide synaptic inputs to motor neurons that potentiate backward movements, exhibited not only an overall reduction in the calcium level increase in nca(lf) and nlf-1 mutants during backing, they also showed a drastically increased frequency of these smaller calcium peaks, averaging ~20 spikes for wild-type animals, ~51 and ~38 spikes for nca(lf) and nlf-1 mutants, respectively, during the 3-min recording ( Supplementary Fig. 9 ; also see Fig. 3c in ref. 37 ). Restoring NLF-1 in premotor interneurons fully restored both the calcium transient size [37] and frequency (data not shown), implying a critical role of premotor interneurons for robust persistent rPSCs. To test this possibility directly, we compared the effect of restoring NCA and NLF-1 in all or subgroups of neurons, in nca(lf) and nlf-1 mutants, respectively, on the presence of persistent rPSCs and sustainability of locomotion. Restoring NCA and NLF-1 panneuronally ( Prgef-1 ) led to a complete restoration of persistent rPSCs ( Fig. 3 ; Supplementary Fig. 8 ), movements with long duration ( Fig. 2 ; Supplementary Fig. 5 ) and a reduction in movements with short duration and directional transition ( Fig. 2c ). Restoring NCA in multiple neurons, which include the entire premotor interneuron network ( Pnmr-1+Plgc-55s ; Methods), led to a robust rescue of motor defects and persistent rPSCs in nca(lf) mutant ( Fig. 2 ; Fig. 3 ). This was in contrast to restoring NCA expression in all excitatory (cholinergic) motor neurons ( Psto-6 ), or in all inhibitory (GABAergic) motor neurons ( Punc-25 ), which were insufficient to rescue above defects in nca(lf) mutants ( Fig. 2 ; Fig. 3 ). These results suggest that premotor interneurons are necessary for generating or maintaining persistent rPSCs, and persistent rPSC-dependent sustention of locomotion. The panneuronal NCA transgene exhibited a slightly stronger rescue effect than the premotor NCA transgene, which may be caused by transgene variability (Methods), and/or, reflect a minor contribution from non-premotor interneurons. 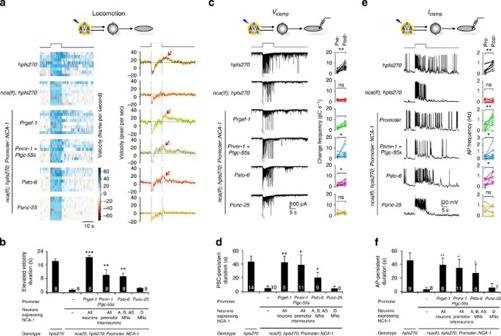Figure 4: Persistent activity correlates with sustained acceleration. (a) Raster plots (left panels) and the mean (right panels) of the instantaneous velocity of directional movement in free-moving animals of indicated genotypes, pre, during and post-10s-blue light stimulation. All animals containedhpIs270where ChR2 was expressed exclusively in AVA among all premotor interneurons (schematic in the upper panel andFig. 1e). Left, each horizontal bar represents the raw data from one recording. Dark colorus present higher velocity. Shaded areas with vertical dashed lines denote the illumination periods.+ and − in the scale bar represents velocity in forward and backward directions, respectively. Right, traces of averaged velocity of each genotype. Arrows denote the velocity post stimulation. Horizontal dashed lines denote the resting velocity before stimulation; the vertical dashed lines denote the illumination periods. (b) Quantification of the duration of elevated velocity after the stimulation. The extended period of acceleration after stimulation was diminished innca(lf)mutants, a deficit that was significantly rescued by restoring NCA-1 expression in all premotor interneurons (Pnmr-1+Plgc-55s), or all excitatory motor neurons (Psto-6). (c) Left panels, representative rPSC traces of the same set of animals as ina, before and after the same stimulation protocol (10-s blue light). Right panels, rPSCs charge frequency before and after the stimulation. Connected lines represent recordings from the same preparation. (d) Quantification of the duration of persistent rPSCs from recordings shown inc. (e,f) Representative traces (e) and quantification (f) of the body wall muscle (BWM) AP firing of the same set of animals pre- and post-10-s blue light stimulation. Muscles were held at −60 mV inVclampand at 0 pA inIclamp, respectively. *P<0.05, **P<0.01, ***P<0.001, againstnca(lf)mutants by the Mann–WhitneyU-test. Error bars, s.e.m. Figure 4: Persistent activity correlates with sustained acceleration. ( a ) Raster plots (left panels) and the mean (right panels) of the instantaneous velocity of directional movement in free-moving animals of indicated genotypes, pre, during and post-10s-blue light stimulation. All animals contained hpIs270 where ChR2 was expressed exclusively in AVA among all premotor interneurons (schematic in the upper panel and Fig. 1e ). Left, each horizontal bar represents the raw data from one recording. Dark colorus present higher velocity. Shaded areas with vertical dashed lines denote the illumination periods.+ and − in the scale bar represents velocity in forward and backward directions, respectively. Right, traces of averaged velocity of each genotype. Arrows denote the velocity post stimulation. Horizontal dashed lines denote the resting velocity before stimulation; the vertical dashed lines denote the illumination periods. ( b ) Quantification of the duration of elevated velocity after the stimulation. The extended period of acceleration after stimulation was diminished in nca(lf) mutants, a deficit that was significantly rescued by restoring NCA-1 expression in all premotor interneurons ( Pnmr-1 + Plgc-55s ), or all excitatory motor neurons ( Psto-6 ). ( c ) Left panels, representative rPSC traces of the same set of animals as in a , before and after the same stimulation protocol (10-s blue light). Right panels, rPSCs charge frequency before and after the stimulation. Connected lines represent recordings from the same preparation. ( d ) Quantification of the duration of persistent rPSCs from recordings shown in c . ( e , f ) Representative traces ( e ) and quantification ( f ) of the body wall muscle (BWM) AP firing of the same set of animals pre- and post-10-s blue light stimulation. Muscles were held at −60 mV in V clamp and at 0 pA in I clamp , respectively. * P <0.05, ** P <0.01, *** P <0.001, against nca(lf) mutants by the Mann–Whitney U -test. Error bars, s.e.m. Full size image nlf-1 mutants exhibited a similar neuronal requirement: a restoration of NLF-1 in the premotor interneuron network ( Pnmr-1+Plgc-55s ) led to a similar degree of restoration of persistent rPSCs ( Supplementary Fig. 8 ) and the sustainability of basal movements, as the panneuronal restoration ( Prgef-1 ) of NLF-1 ( Supplementary Figs 4 and 5 ). Slightly different from the case for NCA, however, was that the restoration of NLF-1 in all excitatory motor neurons ( Psto-6 ) also led to a robust rescue of persistent rPSCs ( Supplementary Fig. 8 ) and some motor defects (for example, directional transition; Supplementary Figs 4b and 5 ). We noted that, unlike the case for premotor interneuron NLF-1, NLF-1 expression in excitatory motor neurons did not fully restore nlf-1 ’s motor defects (for example, backing duration; Supplementary Fig. 5a,b ). Moreover, nlf-1 mutants exhibited a milder reduction of persistent rPSCs when compared with nca(lf) , which coincided with a slightly less severe motor defects than nca(lf) animals [37] . The ability of premotor interneuron-specific restoration of NCA and NLF-1 to rescue persistent rPSCs and locomotion pattern supports a critical role of premotor interneurons in maintaining the persistent motor circuit network activity, which sustains basal locomotion under standard culture conditions. Persistent rPSCs are associated with sustained acceleration Bursts of action potentials induce sustained C. elegans body wall muscle contraction [44] , [48] . The correspondence between persistent rPSCs and post-stimulation action potential bursts indicates that persistent rPSCs are capable of sustaining muscle contraction, and hence are functionally relevant for post-stimulation motor behaviours. To examine this possibility directly, we applied the same photostimulation protocols, which we used to evoke persistent rPSCs in the electrophysiology preparations, to freely moving animals (Methods). Upon ChR2-induced photoactivation of a single pair of premotor interneurons AVA, wild-type animals ( hpIs270 ) responded with an immediate bout of backing ( Fig. 4a ). This is consistent with previous reports, where ChR2-induced activation of a neural network that included premotor interneurons AVA, AVE, AVD and RIM induced immediate backing [52] , [53] . During the sustained stimulation, wild-type animals exhibited a decay of backing velocity that transited into forward movements ( Fig. 4a ). At the end of the stimulation, wild-type animals typically exhibited a velocity higher than that of pre-stimulation, and the acceleration was sustained for ~18 s before returning to the pre-stimulation velocity ( Fig. 4a,b ). Consistent with this motor behaviour, wild-type animals exhibited an increased charge frequency and duration of persistent rPSCs by voltage clamp recording ( Fig. 4c,d ), and an increased frequency and duration of post-stimulation action potential firing by current clamp recording, during the 40-s post-stimulation period ( Fig. 4e,f ). In nca(lf) mutants with hpIs270 , activation of the AVA premotor interneurons induced a bout of backing with a similar velocity as that of wild-type animals ( Fig. 4a ). However, they exhibited a faster decay of backing velocity during sustained stimulation. The velocity returned to the pre-stimulation baseline either during or immediately after the stimulation ( Fig. 4a,b ). Consistent with their inability to exhibit post-stimulation acceleration, these animals did not display increased charge transfer or action potential frequency post-stimulation ( Fig. 4c–f ). These results thus support the physiological correlation between persistent rPSCs and sustained acceleration post-premotor interneuron stimulation. Lastly, when NCA was restored in premotor interneurons ( Pnmr-1 + Plgc-55s ), the post-stimulation responses evoked from the AVA neurons, including the increased velocity ( Fig. 4a,b ), the increased charge transfer, persistent rPSCs and action potential firing ( Fig. 4c–f ), were significantly restored in nca(lf) mutants. This is similar to a critical requirement of NCA in premotor interneurons to sustain spontaneous locomotion ( Fig. 2 ) and persistent rPSCs evoked from multiple premotor interneurons ( Fig. 3 ). Similarly, no rescue was observed when NCA was restored in GABAergic motor neurons ( Punc-25 ). Differing from the case for basal locomotion, however, a restoration of NCA expression in cholinergic motor neurons ( Psto-6 ) also led to a significant rescue of the post-stimulation increase in velocity, charge transfer, persistent rPSCs and action potential firing ( Fig. 4 ), indicating a contribution of the excitatory motor neurons for persistent motor circuit activity under evoked conditions. Together, these results support a critical role of the NCA channel in premotor interneurons to sustain basal locomotion upon stimulation. They also reveal the ability of cholinergic motor neurons in generating or maintaining rPSCs upon strong premotor interneuron stimulation. Persistent neural activity, a sustained circuit output that outlasts the stimuli, underlies working memories and behaviours that require short-term information retention. To date, electrophysiology analyses on both in vivo and in vitro vertebrate preparations have mainly relied on pharmacological interventions to reveal mechanisms for persistent neural activity. Here the advent of optogenetics and improvement in the C. elegans neuromuscular preparation allowed us to document the first observation of such persistent activity. Combining molecular genetics, electrophysiology and quantitative behavioural analyses, we further demonstrate that persistent motor circuit activity is physiologically relevant for sustained locomotion, and it requires a recently discovered sodium leak channel NCA ( Supplementary Table 1 ). These findings testify C. elegans’ suitability as a model to dissect the molecular bases for persistent neural activity. Previous studies have proposed different mechanisms for generating persistent activity: reverberant neural networks that depend on synaptic connections, or, single neurons with intrinsic properties to elicit long-lasting outputs. Because the NCA channel exhibits a prominent functional requirement in premotor interneurons, we tested a possibility that premotor interneuron themselves can generate persistent activity by whole-cell voltage clamp recording of AVA. Upon direct stimulation of AVA by ChR2 ( hpIs270 ), we observed, in three out of four recordings, a post-stimulation discharge increase. These results support AVA’s latent ability to generate persistent neural activity ( Supplementary Fig. 10 ). It should be noted, however, that this result does not exclude the possibility that synaptic connections between AVA and other premotor interneurons account for the observed sustained activity post stimulation. Because AVAs are predominantly postsynaptic to other premotor interneurons, we cautiously favour the possibility that some premotor interneurons such as AVA may generate self-sustained persistent neural activity. How NCA regulates persistent neural activity is unknown. It may activate an unknown CAN channel, or its own conductance accounts for premotor interneuron’s ability to exhibit persistent activity. To our best knowledge, the motor deficits of fainters are unique to mutations in the NCA channel components, suggesting that NCA channel may constitute part of the intrinsic property of AVA to sustain activity post stimulation. The AVA premotor interneurons instruct motor neurons through both gap junctions and chemical synapses. One plausible possibility is that the NCA channel allows AVA to sustain prolonged depolarization and release of neurotransmitters to maintain motor neuron activity post stimulation. NCA thus constitutes an intrinsic ionic conductance of premotor interneurons that potentiates their persistent activity post stimulation. Alternatively, or, in parallel, NCA supports long-lasting post-stimulation activity by potentiating synaptic communications within the premotor interneuron network. While our study consistently pointed to a critical role of premotor interneurons in persistent motor circuit activity, it further revealed an interesting mechanistic difference for sustained motor behaviours under evoked and non-evoked conditions. The premotor interneuron NCA was essential for restoring nca(lf) locomotion in the absence of stimulation. However, upon optogenetic stimulation of premotor interneurons, the loss of persistent motor circuit activity could also be rescued by restoring NCA in either premotor interneurons or their postsynaptic partners, the cholinergic motor neurons. This is in line with a possibility that motor neurons also can generate persistent activity under appropriate activation conditions. An attractive hypothesis is thus that persistent neural activity, which sustains continuous movement, is potentiated through premotor interneurons during spontaneous movements, but when strong stimuli are presented, other components, such as motor neurons, are recruited to prolong the motor system’s persistent firing before returning to its pre-stimulation state. Lastly, a critical contribution of premotor interneurons in sustaining organized motor activity is unlikely unique for C. elegans , but likely a shared mechanism for many motor systems. For example, a brief stimulation of the hindbrain–spinal cord premotor interneurons was sufficient to generate prolonged swimming in frog tadpoles [54] . Optogenetic activation of the excitatory V2a ipsilateral premotor interneurons in the zebrafish larva resulted in a long bout of bursting activity that outlasted the stimulus (see Fig. 2h in ref. 55 ). It would thus be of interest to examine the role of the NCA family sodium leak channel in other motor circuits. Strains All strains were cultured at 22 °C on Nematode Growth Medium (NGM) plates seeded with OP50, unless specified otherwise. The following strains were used in this study: wild-type N2 Bristol unless specified otherwise (see Figure legends), ZM4624 hpIs166 ; ZM6804 hpIs270 , ZM1659 nca-2(gk5);nca-1(gk9) (referred to as nca(lf) in the study), ZM6610 nlf-1(hp428) , ZM4620 nca-2(gk5);nca-1(gk9);hpIs166 , ZM7218 nlf-1(hp428);hpIs166 , ZM7536 nca(lf);hpIs270 . Transgenic animals carrying extrachromosomal arrays ( hpEx lines) were generated by co-injecting an injection marker and a given construct at 5–30 ng μl −1 . Animals carrying transgenes integrated into the C. elegans genome ( hpIs lines) were generated from the indicated hpEx lines by ultraviolet irradiation. All deletion ( gk ) or integrated transgenic ( hpIs ) strains were outcrossed against N2 at least twice beforeanalyses. All strains that contained hpIs166 and hpIs270 were cultured in the dark at 22 °C on NGM plates supplemented with or without ATR as described previously [43] . L4-stage or young adult (24 h post L4) hermaphrodites were used in all experiments. Molecular biology Following constructs were generated, and injected in nlf-1(hp428); hpIs166 , with Podr-1 ::GFP as the co-injection marker, to generate transgenic animals expressing NLF-1 under various neuronal promoters. For nlf-1 neuronal-specific rescue constructs, all neuronal promoters were described in our previous studies [56] . The full-length nlf-1 cDNA clone (pJH2432) was obtained by reverse transcriptase–PCR (RT–PCR) against a mixed-stage C. elegans cDNA library with oligoes OZM2429 aaGGATCCttatgcggcctcgcacgccttacaca and OZM2545 ccGGTACCccctataacaacaacataaatcgaaga , and cloned into pBSK. cDNA sequence was confirmed by sequencing, and used for the following NLF-1 neuronal subtype rescuing experiments. pJH2437, a clone that expresses NLF-1 cDNA under a panneuronal promoter Prgef-1 , followed by unc-54 3-untranslated repeat (UTR), fully rescued the fainter phenotype of nlf-1(hp428) animals. The same cDNA fragment was subsequently subcloned into vectors containing various subtype neuronal promoters and unc-54 3′UTR, pJH2440 ( Pnmr-1 ::NLF-1), pJH3259 ( Plgc-55s ::NLF-1), pJH2439 ( Psto-6 ::NLF-1) and pJH2162 ( Punc-25 ::NLF-1). Information on the Pnmr-1 , Psto-6 and Punc-25 promoter fragments used in this study has been described previously [56] ; Plgc-55s is a smaller fragment from previously described Plgc-55 (corresponding to 120 to +773 nt into the translation initiation site of LGC-55, with the membrane targeting signal (nt +4 to +48) removed 57), which restricts the expression to AVB and a few non-premotor interneurons. Following constructs were generated and injected in nca(lf);hpIs166 or nca(lf);hpIs270 animals with Pmyo-2 ::RFP as the co-injection marker to generate transgenic animals expressing NCA-1::GFP under various neuronal promoters. The panneuronal NCA-1::GFP transgene (pJH3010) was generated by cloning an 8-kb BglII fragment from WRM0613dC08 that contains the N-terminal portion of the nca-1 genomic DNA into the BamHI site of a panneuronal promoter vector pJH625. The panneuronal NCA-1 transgene ( Prgef-1 ::NCA-1::GFP) was generated by co-injecting pJH3010 with a PCR-stitched C-terminal NCA-1::GFP fragment as previously described [33] . The panneuronal promoter was then switched to different neuronal promoters to generate pJH3178 ( Pglc-55s ::NCA-1::GFP), pJH3153 ( Pnmr-1 ::NCA-1::GFP), pJH3107 ( Psto-6 ::NCA-1::GFP) and pJH3152 ( Punc-25 ::NCA-1::GFP). pJH1697 ( Pglr-1 ::ChR2(H134R)::YFP) was generated by swapping of the Cerulean fragment of pJH554 ( Pglr-1 ::Cerulean) with the ChR2(H134R)::YFP fragment from pJH1684 ( Pmec-4 ::ChR2(H134R)::YFP). pJH2690 ( Prig -3::FLFssChR2(H134R)::wCherryex) was generated by ligating the Prig-3 promoter fragment from pJH1968 ( Prig-3 ::UNC-1::UrSL::wCherry) with the FLF-ssChR2(H134R)::wCherryex (ss stands for signal peptide; ex stands for ER export signal) fragment from pJH2654 ( Pnmr-1 ::RF::ssChR2(H134R)::wCherryex). pJH2673 ( Pnmr-1 ::FLP) was generated by ligating the Pnmr-1 promoter fragment from pJH1925 ( Pnmr-1 ::wCherry) with the FLP fragment from pJH2655 ( Pnsy-5 su::FLP::wCherry). Electrophysiology One-day-old adult hermaphrodite C. elegans was dissected as previously described [42] . Briefly, animals were immobilized on Sylgard 184 Silicone Elastomer (Dow Corning)-coated glass coverslips using tissue adhesive glue (Histoacryl Blue, Braun). The curved anterior dorsal side of the animal was dissected using a sharpened tungsten needle. After clearing the viscera by suction through a glass pipette, the cuticle flap was turned and gently glued down using WORMGLU (GluStitch Inc.) to expose the neuromuscular system. The integrity of the anterior ventral body wall muscle and the ventral nerve cord were visually examined via the DIC microscopy, and ventral muscle cells that reside behind the pharynx and before the vulva were patched using fire-polished 4- to 6-MΩ resistant borosilicate pipettes (World Precision Instruments, USA). Membrane currents were recorded in the whole-cell configuration by a Digidata 1440A and a MultiClamp 700A amplifier using the Clampex 10 software, processed with Clampfit 10 (Axon Instruments, Molecular Devices, USA). Data were digitized at 10−20 kHz and filtered at 2.6 kHz. The pipette solution contains (in mM): K-gluconate 115; KCl 25; CaCl 2 0.1; MgCl 2 5; BAPTA 1; HEPES 10; Na 2 ATP 5; Na 2 GTP 0.5; cAMP 0.5; cGMP 0.5, pH7.2 with KOH, ~320 mOsm. The bath solution consists (in mM) of the following: NaCl 150; KCl 5; CaCl 2 5; MgCl 2 1; glucose 10; sucrose 5; HEPES 15, pH7.3 with NaOH, ~330 mOsm. All chemicals were obtained from Sigma. Experiments were performed at room temperature (20−22 °C). Five to seventeen animals were analysed in each experiment. The number of animals for each experiment was specified in Figures and/or Figure legends. Optogenetic stimulation of the dissected hpIs166 and hpIs270 preparation was performed using an LED light apparatus (KSL-70; RAPP OptoElectronic) at a wavelength of 470 nm (8 mW mm −2 ), controlled by the Axon amplifier software. Unless specified otherwise, 10 s pre- and 30–40 s post-stimulation recordings were analysed. We compared the charge frequency before and after stimulation due to the consistent post-stimulation baseline descent observed in wild-type animals. Auto-tracking locomotion analyses A single 12- to 18-h post-L4 stage adult hermaphrodite, maintained on standard culture conditions, was transferred to a 100-mm imaging plate. One minute after the transfer, a 2-min movie of the crawling animal was recorded on a modified Axioskop 2 (Zeiss) equipped with an automated tracking stage MS-2000 (Applied Scientific Instruments), a digital camera (Hamamatsu) and a homemade blue and yellow LED light sources (Thorlabs). The imaging plates were standard NGM plates seeded with a thin layer of OP50 12–14 h before the experiment. Immediately before the transfer of worms, the OP50 lawn was spread evenly across the plate with a sterile bent glass rod. Movements exhibited by C. elegans were recorded using an in-house developed automated tracking programme. All images were captured with a × 10 objective, at 10 frames per second. Data obtained from at least ten animals per genotype, recorded on the same plate and on the same day, were pooled, quantified and compared. Post-imaging analyses utilized an in-house developed ImageJ Plugin [56] , which skeletonizes each image and divides the length of the animal into 33 segments. The centroid of the animal was used to track and calculate the velocity and direction of the animal’s movement between each frame. The percentage of total frames exhibiting pausing, backward or forward backward movement was defined by the centroid position change: between −1 (− was defined as movement towards the tail) and +1 (+ was defined as movement towards the head) pixel per second was defined as pausing, less than −1 pixel per second backward and more than +1 pixel per second as forward movement. To calculate the initiation and duration of movement, we defined that a period of directional movement should have more than two consecutive frames where the centroid moved in the same direction. For optogenetically stimulated behaviour analysis, animals were maintained on standard NGM-OP50 plates supplemented with all- trans retinol. One minute after the transfer of an animal to the imaging plate, a pulse of 10-s 488-nm blue light stimulation was applied to the imaging plate, and the movement of the animal was tracked and recorded for 2.5 min. In Fig. 4a , the instantaneous velocity, with directionality, was plotted over time for each recorded animal; the mean and s.e. were calculated with the pooled data. Statistical analysis Either the Mann–Whitney U -test or two-tailed Student’s t -test was used to compare the difference of most data sets. P <0.05 was considered to be statistically significant (* P <0.05, ** P <0.01, *** P <0.001). Graphing and subsequent analysis were performed with Igor Pro (WaveMetrics), Clampfit (Molecular Devices), Image J (National Institutes of Health), R ( http://www.R-project.org ) and Excel (Microsoft). Unless specified otherwise, each recording trace was obtained from a different animal. Data were presented as the mean±s.e.m. How to cite this article: Gao, S. et al . The NCA sodium leak channel is required for persistent motor circuit activity that sustains locomotion. Nat. Commun. 6:6323 doi: 10.1038/ncomms7323 (2015).